Microfluidic platform for the quantitative analysis of leukocyte migration signatures Leukocyte migration into tissues is characteristic of inflammation. It is usually measured in vitro as the average displacement of populations of cells towards a chemokine gradient, not acknowledging other patterns of cell migration. Here, we designed and validated a microfluidic migration platform to simultaneously analyse four qualitative migration patterns: chemoattraction, -repulsion, -kinesis and -inhibition, using single-cell quantitative metrics of direction, speed, persistence and fraction of cells responding. We find that established chemokines, complement component 5a and IL-8 induce chemoattraction and repulsion in equal proportions, resulting in the dispersal of cells. These migration signatures are characterized by high persistence and speed and are independent of the chemokine dose or receptor expression. Furthermore, we find that twice as many T lymphocytes migrate away than towards stromal cell-derived factor 1 and their directional migration patterns are not persistent. Overall, our platform helps discover migratory signature responses and uncovers an avenue for precise characterization of leukocyte migration and therapeutic modulators. The migration of leukocytes into tissues is characteristic of inflammation [1] , [2] and is tightly controlled by soluble [3] , [4] , [5] and immobilized chemical gradients [6] . Migratory responses induced by chemical cues are traditionally classified into one of the four different patterns that include directional migration towards a secreted protein gradient (chemoattraction) [4] , [5] , [6] , migration in random directions (chemokinesis) [7] , migration away from a source (chemorepulsion) [8] , [9] and reduced migration in any direction (chemoinhibition). However, our ability to characterize these migration patterns is poor in standard migration assays. For example, Boyden chambers [10] , Dunn and Zigmond chambers [11] , [12] , micropipette techniques [13] and most microfluidic-based assays [14] , [15] , [16] , [17] , [18] have significant limitations in quantifying the dynamic nature of the migration process, and typically only monitor a single averaged pattern. The Boyden chamber can be used to directly assess population-averaged migration in one direction (chemoattraction) but can only indirectly assess other patterns of migration (for example, by comparing at least four measurements in a ‘checkerboard’ assay [10] ). It also lacks single-cell resolution, and cannot identify heterogeneous migratory patterns within subsets of leukocytes. The Dunn and Zigmond chambers and micropipette techniques allow for single-cell resolution [11] , [12] , [13] ; however, the ability to differentiate among different migration patterns is hampered by large variations in speed and directionality, which is typical for cells migrating on flat surfaces [19] . Until recently, microfluidic assays have focused on technology, such as controlling the shape and stability of chemical gradients [17] , competing gradients [20] or on-chip neutrophil purification from whole-blood samples [18] , [21] . However, the large variations in speed and directionality during leukocyte chemotaxis on flat surfaces in microfluidic devices limit precision for studies that require quantification of leukocyte migration [15] , [16] , [17] , [18] . Newer microfluidic devices that confine moving leukocytes within small channels circumvent these problems and enable significantly higher precision measurements of leukocyte migration [14] , [22] , [23] , [24] . Microfluidic devices enabled our group to define a normal range of human neutrophil velocity in healthy individuals [14] and helped optimize a treatment that restores defective neutrophil directionality following burn injuries [22] . However, like other chemotaxis assays, these devices were designed only to measure chemoattraction and ignored other cell migration patterns. In this study, we design and validate a microfluidic device that employs two large-scale arrays of microchannels to facilitate the quantification of leukocyte migration both towards and away from chemical gradients. The device ensures that a precise number of cells are exposed to identical conditions at the initiation of the experiment and enables us to identify specific leukocyte migration signatures in response to well-established chemokines. Whereas the neutrophil chemoattractants fMet-Leu-Phe (fMLP) and leukotriene B4 (LTB4) induce chemoattraction that is fast and persistent, we show that interleukin-8 (IL-8) and complement component 5a (C5a) [25] , [26] induce both chemoattraction and repulsion in equal proportions with high migratory persistence and speed. These effects are not dose-, receptor- or subset dependent, but rather appear to be cell intrinsic. Similarly, stromal cell-derived factor 1 (SDF-1) acts on lymphocytes to induce both attraction and repulsion, although twice as many lymphocytes migrate in a chemorepulsive rather than in a chemoattractant manner and directional migration patterns are not persistent. Furthermore, we show that the neutrophil inhibitor Slit2 alters the size of migrating subpopulations of neutrophils without changing their overall migration patterns. The data presented in this report provides a quantitative analysis of leukocyte migration patterns not previously defined in vitro using traditional techniques. We suggest that multiparameter assessment of migration has great potential for functional mechanistic analyses, and is critical for the optimal design of anti-inflammatory agents. Microfluidic device for evaluation of leukocyte migration We designed a microfluidic device in which precise numbers of leukocytes are reproducibly loaded and uniformly distributed into a central main channel with cell traps. After loading, the cells leave the traps and migrate into side channels (6 × 6 μm or 50 × 6 μm for neutrophils and 10 × 6 μm for lymphocytes). Half of the channels lead into an array of chemokine reservoirs (on one side of the main channel) and half (on the opposite side) lead into a channel with buffer alone ( Fig. 1a and Supplementary Fig. 1A ). This design allows for the formation of two spatial chemokine gradients on each side of the central main channel, one with an increasing gradient towards the chemokine and the other with a decreasing concentration gradient towards the channel with buffer. We tested the stability of chemical gradients within the device channels, and found that they remained constant for~12 h in both 6 and 10 μm channels and for~4 h in 50 μm channels ( Fig. 1b ). The simultaneous presence of the two gradients enables quantitative measurements at single-cell resolution of migration both towards and away from gradients, from the same initial condition for all cells in a given population. 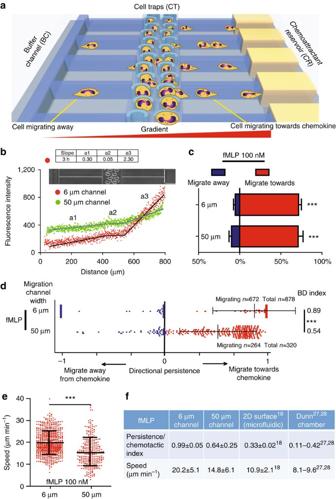Figure 1: Measuring attraction, repulsion, kinesis and inhibition during leukocyte responses to chemical gradients. (a) Cell migration in mechanically confined spaces can be characterized in relation to the direction of the chemical gradients and quantified for speed, directionality and persistence. Cells loaded in the cell traps (CT) can either migrate towards or away from the chemokine gradient. (b) Characterization of the stable chemical gradients that can be established in the device. Fluorescein labelled dextran of 10 kDa was used. After 3 h, a steep gradient is preserved in 6 μm channels, while in 50 μm channels a shallower gradient is preserved. a1 represents the migration channel from the buffer channel (BC) towards the cell-loading chamber, a2 the cell-loading chamber and a3 the migration channel from cell-loading chamber towards the chemokine reservoir. (c) Percentage of human neutrophils loaded in the migration channel that migrate towards or away from fMLP in 6 and 50 μm wide migration channels. Neutrophils migrate in significantly greater numbers towards fMLP than away from it (***P<0.001, Student’st-test). Combined data fromn=3 independent experiments. (d) Scatterplot of migratory persistence of human neutrophils towards and away from a gradient of fMLP in 6 and 50 μm migration channels. The BD index combines persistence and directionality in one parameter and is significantly higher in narrow (6 μm) channels (***P<0.001, Mann–Whitney test). Bars represent mean±s.d. (e) Migratory speed of neutrophils migrating towards fMLP in 6 and 50 μm wide migration channels. Neutrophils migrate significantly faster towards fMLP in 6 μm than in 50 μm channels (***P<0.001, Student’st-test). Bars represent mean±s.d. (f) Effect of migration channel width on migratory persistence and speed of cells migrating towards fMLP. Comparison between the bi-directional microfluidic device and established two-dimensional microfluidic devices and Dunn chambers18,27,28. A total of 878 cells were analysed in 6 μm channels (672 migrated); 320 (264 migrated) in 50 μm channels,n=3. Figure 1: Measuring attraction, repulsion, kinesis and inhibition during leukocyte responses to chemical gradients. ( a ) Cell migration in mechanically confined spaces can be characterized in relation to the direction of the chemical gradients and quantified for speed, directionality and persistence. Cells loaded in the cell traps (CT) can either migrate towards or away from the chemokine gradient. ( b ) Characterization of the stable chemical gradients that can be established in the device. Fluorescein labelled dextran of 10 kDa was used. After 3 h, a steep gradient is preserved in 6 μm channels, while in 50 μm channels a shallower gradient is preserved. a1 represents the migration channel from the buffer channel (BC) towards the cell-loading chamber, a2 the cell-loading chamber and a3 the migration channel from cell-loading chamber towards the chemokine reservoir. ( c ) Percentage of human neutrophils loaded in the migration channel that migrate towards or away from fMLP in 6 and 50 μm wide migration channels. Neutrophils migrate in significantly greater numbers towards fMLP than away from it (*** P <0.001, Student’s t- test). Combined data from n =3 independent experiments. ( d ) Scatterplot of migratory persistence of human neutrophils towards and away from a gradient of fMLP in 6 and 50 μm migration channels. The BD index combines persistence and directionality in one parameter and is significantly higher in narrow (6 μm) channels (*** P <0.001, Mann–Whitney test). Bars represent mean±s.d. ( e ) Migratory speed of neutrophils migrating towards fMLP in 6 and 50 μm wide migration channels. Neutrophils migrate significantly faster towards fMLP in 6 μm than in 50 μm channels (*** P <0.001, Student’s t- test). Bars represent mean±s.d. ( f ) Effect of migration channel width on migratory persistence and speed of cells migrating towards fMLP. Comparison between the bi-directional microfluidic device and established two-dimensional microfluidic devices and Dunn chambers [18] , [27] , [28] . A total of 878 cells were analysed in 6 μm channels (672 migrated); 320 (264 migrated) in 50 μm channels, n =3. Full size image fMLP induces bi-directional migratory patterns in HL-60 cells To validate the device, we first characterized the migratory patterns of a clonal population of HL-60 cells in response to fMLP gradients (maximum concentration, 100 nM). Using speed and directional persistence (DP—see Methods section, Supplementary Fig. 1C ), we divided individual cells into three groups 1) high persistence (DP (0.66–1)), 2) medium persistence (DP (0.33–0.66)), and 3) low persistence (DP (0–0.33)), see Supplementary Fig. 1C–F . For HL-60 cells that respond to fMLP gradients, the largest cluster comprises cells that migrate with high persistence towards the chemoattractant (~67% of all migrating cells, DP (0.66–1), Supplementary Fig. 1E ). The second largest cluster is that of cells that migrate towards the chemoattractant with low persistence, meaning they eventually reverse migrate back to their initial starting position (~13% cells, DP<0.33). A cluster of comparable size comprises cells that migrate in a random manner away from fMLP with low DP (~10% cells, −0.33<DP≤0) and a smaller cluster of HL-60 cells in the device were found to migrate away from fMLP with high DP (~4%, −1≤DP ≤−0.66). Overall, these results highlight the known, dominant function of fMLP as a promigratory chemoattractant. Nevertheless, our findings also demonstrate that significant numbers of clonal HL-60 cells migrate in a random and/or repulsed manner. Higher migratory persistence in narrow migration channels We compared the migratory response of human neutrophils with fMLP gradients in narrow 6 μm and wide 50 μm channels ( Supplementary Movies 1 and 2 ). We found that the numbers and proportions of migrating neutrophils are comparable in narrow and wide channels. In 6 μm channels, a total of 71.5±3.8% neutrophils migrated towards fMLP and 5.4±1.7% migrated away from it, whereas in 50 μm channels, chemoattraction was noted in 71.2±3.4% and chemorepulsion in 9.7±2.8% of the neutrophils; a total of 23% cells (in 6 μm) and 20% cells (in 50 μm) did not migrate, respectively ( Fig. 1c ). Cell movement towards fMLP was significantly more persistent in 6 μm channels, where 90% of moving neutrophils migrated with maximum DP (DP=1) and with a high bi-directional index (BD index=0.89). In the wider 50 μm channels, we found that cells failed to achieve maximal DP and the BD index was significantly reduced (BD index=0.54) compared to migration in 6 μm channels ( Fig. 1d , P <0.001). As illustrated in Fig. 1e , migratory speed was also significantly faster in 6 μm channels (20.2±5.1 μm min −1 compared to 14.8±6.1 μm min −1 , P <0.001). The trend for reduced DP and slower speed with decreasing mechanical confinement is further supported by the evaluation of neutrophil migration measurements in two-dimensional surface microfluidic devices and traditional Dunn chambers ( Fig. 1f ). In these assays, neutrophil migration takes place on flat surfaces, guided exclusively by chemical gradients and no mechanical restrictions, resulting in low migratory persistence (0.11–0.42 on flat surfaces versus 0.99 in 6 μm channels) and speed (8.1–10.9 μm min −1 versus 20.2 μm min −1 in 6 μm channels) [18] , [27] , [28] . Thus, confinement of cells within narrow channels that have a cross sectional area comparable to extracellular matrix [29] is similar to that of leukocytes following paths of least resistance in tissues [30] and is associated with a fast and persistent migratory response. In separate experiments, we compared the response of human neutrophils to fMLP and LTB4. We observed that 76.9±3.9% and 68.9±9.7% of human neutrophils migrated to fMLP and LTB4, respectively. Of the motile neutrophils, 93% and 89% migrated towards each chemoattractant with high DP (DP>0.66, Fig. 2a–c , P <0.01). We found that the average DP towards LTB4 decreases from 0.99±0.09 to 0.74±0.19 ( P <0.001) and the average BD index decreases from 0.79±0.56 to 0.70±0.28 ( P <0.001) in wider versus narrower channels ( Supplementary Fig. 3 ). Moreover, we observed differences in the neutrophil migration patterns after neutrophils exit the wider versus narrower migration channels and enter the chemokine reservoirs. While the neutrophils migrating through wide migratory channels continue to migrate inside the chemokine reservoirs ( Supplementary Movies 1 and 2 ), the neutrophils exiting narrow channels stop migrating quickly after entering. This phenomenon could be explained by the differences in the gradient slope inside the chemokine reservoirs. The flux of chemokine from the reservoir through the wider migration channels (300 μm 2 crosssection) can be almost an order of magnitude larger than in narrower migration channels (36 μm 2 ). This larger gradient inside the reservoirs connected to wider versus narrower channels might allow for ongoing migration within reservoirs. 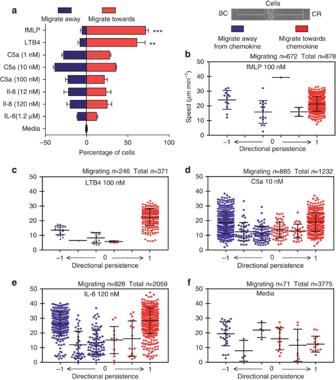Figure 2: Migration patterns of human neutrophils in response to fMLP, LTB4, C5a and IL-8. (a) Percent of human neutrophils that migrate towards or away from fMLP, LTB4, C5a and IL-8 at different concentrations. Human neutrophils migrate in significantly greater numbers towards fMLP and LTB4 than away (P<0.001 andP<0.01 respectively, Student’st-test). Human neutrophils migrate towards and away from C5a and IL-8 in similar proportions. Directionality and speed of neutrophils in response to (b) fMLP (100 nM,n=4), (c) LTB4 (100 nM,n=3), (d) C5a (10 nM,n=4), (e) IL-8 (120 nM,n=4), and (f) cell culture media alone (n=6). Bars represent mean±s.d. For all graphs red colour represents migration towards a chemokine and blue represents migration away from a chemokine. Figure 2: Migration patterns of human neutrophils in response to fMLP, LTB4, C5a and IL-8. ( a ) Percent of human neutrophils that migrate towards or away from fMLP, LTB4, C5a and IL-8 at different concentrations. Human neutrophils migrate in significantly greater numbers towards fMLP and LTB4 than away ( P <0.001 and P <0.01 respectively, Student’s t- test). Human neutrophils migrate towards and away from C5a and IL-8 in similar proportions. Directionality and speed of neutrophils in response to ( b ) fMLP (100 nM, n =4), ( c ) LTB4 (100 nM, n =3), ( d ) C5a (10 nM, n =4), ( e ) IL-8 (120 nM, n =4), and ( f ) cell culture media alone ( n =6). Bars represent mean±s.d. For all graphs red colour represents migration towards a chemokine and blue represents migration away from a chemokine. Full size image C5a and IL-8 induce random neutrophil migration patterns We next compared the patterns of migration of human neutrophils to well-established chemoattractants IL-8 and C5a [25] , [26] , [31] , [32] , [33] . While previous studies have defined average population based responses to these chemokines, we found that each chemokine elicits a distinct migration signature, defined by direction, speed and DP of individual cells ( Fig. 2 ; Table 1 ). We found that the response of human neutrophils to IL-8 (120 nM) and C5a (10 nM) is more heterogeneous, with two distinct subpopulations of comparable size moving with high persistence towards and away from the gradient ( Supplementary Movie 3 ). A total of 35.8±1.2% of neutrophils migrated towards and 38.4±3.0% migrated away from the C5a gradient. Similarly, 25.4±5.2% of neutrophils migrated towards and 19.9±3.6% migrated away from the IL-8 gradient ( Fig. 2a ). Neutrophils that respond to C5a also include a significant fraction of cells (5–10%) that migrate with low persistence (DP<0.33) in both directions ( Fig. 2d ). Speed was found to be similar in the two populations responding to C5a at 17.9±6.6 μm min −1 (attracted subpopulation) and 16.6±7.8 μm min −1 (repelled subpopulation, Supplementary Fig. 2A ). Furthermore, we found that neutrophils migrated with marked persistence towards IL-8, but had a lower persistence when migrating away from IL-8 (DP: 0.94 versus −0.73 P <0.001). Migratory speed of the attracted population in response to IL-8 was higher (27.6±9.4 μm min −1 ) than that of the repelled population (22.0±10.4 μm min −1 ) ( P <0.001). In control experiments using media only, a small number of human neutrophils migrated and their directionality and DP were heterogeneous ( Fig. 2f ). Table 1 Summary of the quantitative analysis of cell migration patterns in this study. Full size table Effect of chemokine concentration on the migratory signatures We next investigated concentration-dependent changes in migration patterns in response to IL-8 and C5a. As illustrated in Fig. 2a , we found that changes in chemokine concentrations primarily affect the size of the migrating population and had no effect on directionality. Increasing IL-8 concentrations from 120 nM to 1.2 μM resulted in a 50% decrease in the total fraction of migrating cells, while increasing C5a concentrations from 10 to 100 nM resulted in a 30% reduction of responding cells. We also found that the highest concentrations of IL-8 (1.2 μM) and C5a (100 nM) reduced migratory speed in both the attracted and repelled subpopulations (as compared with 120 nM IL-8 and 10 nM C5a ( Table 1 )). Reducing the concentration of C5a to 1 nM also decreased the fraction of migrating cells, an effect not seen with lower IL-8 concentration (12 nM, Fig. 2a ). Interestingly the migratory speed and DP were both significantly higher in response to the lowest concentration of C5a (1 nM versus 10 and 100 nM, P <0.001 and P <0.05, respectively). Donor variability and neutrophil migration patterns We found a large variability in the response rates of neutrophils to IL-8 in blood obtained from different volunteer donors, and this difference was not observed with C5a and fMLP. A variety index, defined as the ratio between sample s.d. and sample mean, was ~12-fold higher for IL-8 than for C5a, and approximately fourfold higher for IL-8 than for fMLP ( Supplementary Fig. 2B ). We speculated that this variability may be related to the heterogeneity of IL-8 receptor expression and/or IL-8 signalling responses within leukocytes, or it may be related to wide differences in the circulating levels of IL-8 in healthy donors [34] . Nevertheless, we did not find any difference in BD migration signatures of neutrophils in response to IL-8 between individual blood donors. Effect cell confinement on bi-directional migration patterns As shown in Table 2 and Supplementary Fig. 3A , we found that BD migratory patterns are not affected by migratory channel width. Neutrophils migrate in approximate equal proportions both towards and away from C5a and IL-8 in both narrow 6 μm wide and in 50 μm wide channels ( Supplementary Movies 3 and 4 ). However, the migratory persistence and speed of migrating neutrophils was significantly lower in the 50 μm wide channels compared with the 6 μm channels ( P <0.001, Fig. 1f ; Supplementary Fig. 3B,C ). DP also decreases significantly ( P <0.001) both towards and away from both IL-8 and C5a in 50 μm wide channels ( Table 2 ). As shown in Supplementary Fig. 3C , the overall migration pattern (BD index) in wider channels does not change for C5a but the pattern becomes more random (lower BD index) in response to IL-8 (BD index from 0.20±0.88 to −0.02±0.37, P <0.001). Table 2 Summary of the quantitative analysis of cell migration patterns of human neutrophils in 50 μm wide migration channels. Full size table Effect of receptor expression on bi-directional migration We also wished to determine if the chemoattraction and chemorepulsion response(s) of neutrophils in IL-8 and C5a gradients are associated with cellular phenotype. Fluorescence-assisted cell-sorted IL-8R hi -expressing (CXCR1/CD181) (highest 25%ile) and IL-8R lo -expressing (lowest 25%ile) cells were evaluated for their respective migratory response to IL-8 ( Fig. 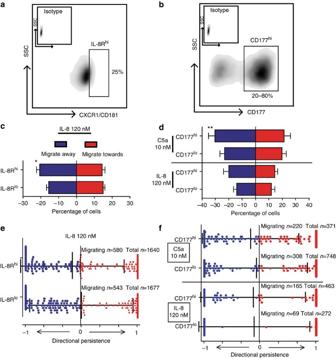Figure 3: Migratory patterns of neutrophil subpopulations. (a) Human neutrophils were fluorescence-activated cell sorted in two groups: highest and lowest quartile expressing IL-8R (CXCR1, CD181). (b) Subpopulations of neutrophils expressing high levels of CD177 (CD177hi) were sorted and compared to CD177locells. The percentage of CD177hicells ranged from 20–80% of total neutrophils. (c) IL-8Rhiand IL-8Rlo-expressing neutrophils show bi-directional migration patterns, but greater numbers of IL-8Rhicells migrate away than towards IL-8 (*P<0.05, Student’st-test). (d) Both CD177hiand CD177locells migrate in a bi-directional manner in response to C5a or IL-8. Greater numbers of CD177hicells migrate in response to C5a versus CD177locells (P=0.06). Higher numbers of CD177hicells migrate away versus towards C5a (**P<0.01, Student’st-test). (e) Migratory patterns of IL-8Rhiand IL-8Rloneutrophils in an IL-8 gradient; no difference was found in DP. Bars represent mean and s.d. of BD index. (f) Migratory persistence of neutrophil subpopulations towards and away from a gradient of IL-8 and C5a. There is no difference in migration patterns of the subpopulations. Bars represent mean±s.d. Data fromn=3 independent experiments. Number of cells analysed: IL-8Rhi, 580 migrating cells; IL-8Rlo, 543 cells; CD177hiC5a, 220 cells; CD177loC5a, 308 cells; CD177hiIL-8, 165 cells; CD177loIL-8, 69 cells. 3 ; Table 3 ). We found that both groups responded with a similar pattern and displayed bi-directional migratory behaviour. Similar numbers of IL-8R hi and IL-8R lo cells responded to IL-8 (~35% versus ~31%, respectively). Nevertheless, the IL-8R hi neutrophils showed a significant bias for migrating away from IL-8 (20.8±2.1% away versus 14.5±1.6% towards, P <0.05). IL-8R lo neutrophils migrated in equal proportions in both directions (15.1±1.1% towards versus 16.2±1.1% away from IL-8). We did not find significant differences in DP and speed between the two subpopulations ( Supplementary Fig. 4A,B ). Figure 3: Migratory patterns of neutrophil subpopulations. ( a ) Human neutrophils were fluorescence-activated cell sorted in two groups: highest and lowest quartile expressing IL-8R (CXCR1, CD181). ( b ) Subpopulations of neutrophils expressing high levels of CD177 (CD177 hi ) were sorted and compared to CD177 lo cells. The percentage of CD177 hi cells ranged from 20–80% of total neutrophils. ( c ) IL-8R hi and IL-8R lo -expressing neutrophils show bi-directional migration patterns, but greater numbers of IL-8R hi cells migrate away than towards IL-8 (* P <0.05, Student’s t- test). ( d ) Both CD177 hi and CD177 lo cells migrate in a bi-directional manner in response to C5a or IL-8. Greater numbers of CD177 hi cells migrate in response to C5a versus CD177 lo cells ( P =0.06). Higher numbers of CD177 hi cells migrate away versus towards C5a (** P <0.01, Student’s t- test). ( e ) Migratory patterns of IL-8R hi and IL-8R lo neutrophils in an IL-8 gradient; no difference was found in DP. Bars represent mean and s.d. of BD index. ( f ) Migratory persistence of neutrophil subpopulations towards and away from a gradient of IL-8 and C5a. There is no difference in migration patterns of the subpopulations. Bars represent mean±s.d. Data from n =3 independent experiments. Number of cells analysed: IL-8R hi , 580 migrating cells; IL-8R lo , 543 cells; CD177 hi C5a, 220 cells; CD177 lo C5a, 308 cells; CD177 hi IL-8, 165 cells; CD177 lo IL-8, 69 cells. Full size image Table 3 Summary of the quantitative analysis of cell migration patterns of different human neutrophil subpopulations. Full size table We also compared the migration response(s) of the CD177 (NB1) [35] expressing neutrophil subpopulation to C5a and IL-8. While the bi-directional migration pattern was present in both CD177 hi and CD177 lo populations, we found that a greater number of CD177 hi cells migrate away than towards C5a (30.3±4.9% away versus 21.6±4.6% towards, P <0.01, Fig. 3d ). CD177 hi cells did not show a statistically significant migratory bias towards or away from IL-8. In contrast, CD177 lo cells migrated in equal proportions both towards and away from either C5a or IL-8. Furthermore, we did not find differences in speed and DP between CD177 hi and CD177 lo populations ( Fig. 3f ; Supplementary Fig. 4C–F ; Table 3 ). Overall, our measurements indicate that regardless of chemokine receptor expression and subpopulation, neutrophils respond in a bi-directional migration pattern to C5a and IL-8. Migration of T lymphocytes in response to SDF-1 We next examined the patterns of CD3+ T lymphocyte migration in response to SDF-1. In the presence of 10 μg ml −1 SDF-1, 39.0±4.5% of the T cells migrated, with twice as many cells migrating away than towards the SDF-1 gradient (25.7±3.1% versus 13.3±2.0%; P <0.001; Fig. 4a ). We observed that the migratory patterns of T lymphocytes are predominantly non-persistent in as much as ~90% of the cells migrating towards and ~70% of the cells migrating away from SDF-1 change their direction at least once during each migration assay. Only 1.4% of the CD3+ T cells migrate with high persistence towards and 4.7% migrate with high persistence away from SDF-1 ( Fig. 4b ). However, the cells migrating away from SDF-1 move faster than cells migrating towards SDF-1 ( Fig. 4d , P <0.001). We did not observe any dominant chemoattractant effect of lower concentrations of SDF-1 (100 ng ml −1 ). These results clearly demonstrate that SDF-1 has an overall dispersive and chemorepulsive effect on a heterogeneous population of T lymphocytes. 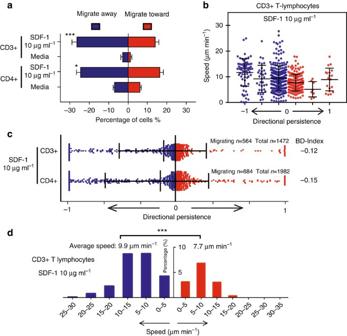Figure 4: Migration of human T lymphocytes in response to SDF-1. (a) Percentage of human T lymphocytes migrating towards or away from SDF-1 (10 μg ml−1) and media (control) Significantly greater numbers of T cells (both pooled CD3+ and CD4+ cells) migrate away from SDF-1 than towards it (***P<0.001 and *P<0.05 respectively, Student’st-test). (b) Distribution of speed and BD index of human CD3+ T lymphocytes in response to SDF-1 (10 μg ml−1). Average persistence of the cells migrating towards and away from SDF-1 is 0.15 and 0.27, respectively. Only ~1.2% of the lymphocytes migrated persistently towards SDF-1, while ~4.7% of the lymphocytes in the device migrated away from SDF-1 with high persistence. (c) Distribution of BD index of T-cell subpopulations. Persistence is very low in all subgroups. (d) Histogram of speed of human CD3+ T lymphocytes in response to 10 μg ml−1SDF-1 in both directions (total 564 cells analysed: 368 repelled cells and 196 attracted cells). Bars represent mean±s.d. Graphs represent combined data ofn=3 independent experiments. Figure 4: Migration of human T lymphocytes in response to SDF-1. ( a ) Percentage of human T lymphocytes migrating towards or away from SDF-1 (10 μg ml −1 ) and media (control) Significantly greater numbers of T cells (both pooled CD3+ and CD4+ cells) migrate away from SDF-1 than towards it (*** P <0.001 and * P <0.05 respectively, Student’s t- test). ( b ) Distribution of speed and BD index of human CD3+ T lymphocytes in response to SDF-1 (10 μg ml −1 ). Average persistence of the cells migrating towards and away from SDF-1 is 0.15 and 0.27, respectively. Only ~1.2% of the lymphocytes migrated persistently towards SDF-1, while ~4.7% of the lymphocytes in the device migrated away from SDF-1 with high persistence. ( c ) Distribution of BD index of T-cell subpopulations. Persistence is very low in all subgroups. ( d ) Histogram of speed of human CD3+ T lymphocytes in response to 10 μg ml −1 SDF-1 in both directions (total 564 cells analysed: 368 repelled cells and 196 attracted cells). Bars represent mean±s.d. Graphs represent combined data of n =3 independent experiments. Full size image We also evaluated the chemoattractive or chemorepulsive migratory signature patterns within CD4+ T cells. As shown in Fig. 4a we found that CD4+ T cells are repelled by SDF-1 in greater numbers (24.4±2.5%) compared to those responding by chemoattraction (16.4±2.5%, P <0.05; Supplementary Movie 5 ). The overall migratory characteristics of pooled CD3+ and CD4+ T cells were very similar (CD3 BD index -0.12, CD4 BD index -0.15, Fig. 4c ; Table 1 ). Collectively, our results indicate that low persistent attraction and repulsive migratory signatures may be a general feature of T cell motility in response to SDF-1. Slit2 inhibits neutrophil chemotaxis to fMLP In a final series of experiments, we wished to validate our microfluidic device for the analysis of anti-inflammatory agents. In these assays, we used Slit2 as a prototype inhibitor of neutrophil migratory responses [36] , [37] , [38] . As illustrated in Fig. 5a , Slit2 (5 μg ml −1 ) reduced the fraction of human neutrophils migrating towards fMLP (100 nM) by approximately threefold (from 74% of cells migrating to 23%, P <0.001). Similarly, we evaluated the effect of Slit2 on the migration of the clonal HL-60 cell line and found that its inhibitory effect was concentration dependent ( Fig. 5 ). Lower numbers of cells migrated at higher concentrations of Slit2 ( P <0.05). Slit2 (1.5 μg ml −1 ) reduced the number of HL-60 cells that migrate towards fMLP (100 nM) by approximately threefold (from 40% to 11%, P <0.01, Fig. 5b ). Slit2 did not reduce the persistence of migrating neutrophils, but it slightly decreased the BD index of migrating HL-60 cells from 0.63±0.57 to 0.39±0.68 ( P <0.001, Fig. 5c,d ). In control experiments, where Slit2 was present in media alone, a migratory response was evident only in 0.8±0.7% of human neutrophils and 12.1±3.4% of HL-60 cells. 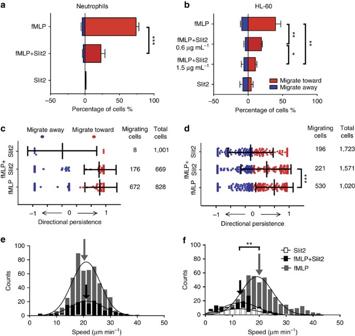Figure 5: Inhibitory effect of Slit2 on fMLP-induced human neutrophil and HL-60 migration. Percentage of (a) human neutrophils and (b) HL-60 cells that migrate towards or away from fMLP in the absence or presence of Slit2 (n=3 andn=4 independent experiments, respectively). For both cell types Slit2 significantly inhibits fMLP-induced migration (**P<0.01 and ***P<0.001 respectively, Student’st-test). (c,d) Migratory persistence of human neutrophils (c) is not affected by Slit2 (fMLP BD index=0.89, fMLP+Slit2 BD index=0.84). (d) DP of migrating HL-60 cells is decreased by Slit2 (fMLP BD index=0.63, fMLP+Slit2 BD index=0.39; ***P<0.001, Mann–Whitney test). Bars represent mean and s.d. of BD index. Speed of (e) neutrophils and (f) HL-60 migrating towards fMLP with or without Slit2 (arrows indicate the mean speed. Slit2 decreases migratory speed of HL-60 cells from 20.7±7.1 μm min−1to 12.8±5.9 μm min−1(P<0.01, Student’st-test). Colours are: grey, fMLP alone; black, fMLP and Slit2; white, Slit2 alone. Bars represent mean±s.d. Combined data ofn=4 (neutrophils) andn=3 (HL-60) independent experiments is shown. For neutrophils and fMLP, a total of 672 migrating out of 828 total cells were analysed, fMLP+Slit (176 migrating/669 total), HL-60 (fMLP 530/1020), fMLP+Slit (221/1571). Figure 5: Inhibitory effect of Slit2 on fMLP-induced human neutrophil and HL-60 migration. Percentage of ( a ) human neutrophils and ( b ) HL-60 cells that migrate towards or away from fMLP in the absence or presence of Slit2 ( n =3 and n =4 independent experiments, respectively). For both cell types Slit2 significantly inhibits fMLP-induced migration (** P <0.01 and *** P <0.001 respectively, Student’s t- test). ( c , d ) Migratory persistence of human neutrophils ( c ) is not affected by Slit2 (fMLP BD index=0.89, fMLP+Slit2 BD index=0.84). ( d ) DP of migrating HL-60 cells is decreased by Slit2 (fMLP BD index=0.63, fMLP+Slit2 BD index=0.39; *** P <0.001, Mann–Whitney test). Bars represent mean and s.d. of BD index. Speed of ( e ) neutrophils and ( f ) HL-60 migrating towards fMLP with or without Slit2 (arrows indicate the mean speed. Slit2 decreases migratory speed of HL-60 cells from 20.7±7.1 μm min −1 to 12.8±5.9 μm min −1 ( P <0.01, Student’s t- test). Colours are: grey, fMLP alone; black, fMLP and Slit2; white, Slit2 alone. Bars represent mean±s.d. Combined data of n =4 (neutrophils) and n =3 (HL-60) independent experiments is shown. For neutrophils and fMLP, a total of 672 migrating out of 828 total cells were analysed, fMLP+Slit (176 migrating/669 total), HL-60 (fMLP 530/1020), fMLP+Slit (221/1571). Full size image We also found that only ~20% of all human neutrophils respond to fMLP within the first 30 minutes. On the other hand, ~65% of HL-60 cells started to migrate within the first 30 min after exposure to fMLP. We observed that Slit2 did not delay the initiation of the neutrophil and HL-60 migratory response to fMLP ( Supplementary Fig. 5A,B ). Also, we observed that Slit2 did not alter the migratory speed of neutrophils ( Fig. 5e and Supplementary Fig. 5C ), but it reduced the migratory speed of HL-60 cells from 20.7±7.1 μm min −1 to an average of 12.8±5.9 μm min −1 ( P <0.01) ( Fig. 5f and Supplementary Fig. 5D ). Overall, these data demonstrate that Slit2 decreases the size of the chemotactic population of human neutrophils, but it does not decrease the initiation of the migratory response, the migratory speed or persistence. This signature effect of Slit2 may have important implications for its development as an anti-inflammatory therapeutic. In this study, we define a new paradigm, whereby individual chemokines elicit distinct signature migratory responses in different leukocyte populations. We show that typical leukocyte migratory responses are the summation of qualitative migratory patterns including attraction, repulsion, kinesis and inhibition. We quantify these patterns using four metrics: (a) percentage of cells migrating in response to a chemokine, (b) directionality, (c) speed, and (d) persistence of migration and we use these metrics to quantify migration signatures with higher precision. By enabling precise, quantitative studies of cell migration, our microfluidic platform creates opportunities to design novel anti-inflammatory agents that target specific migration patterns. Key features in the design of our device enable high precision characterization of cell migration both towards and away from chemical gradients. Cells migrate into side channels from predefined locations and at predefined numbers. The gradient characteristic is defined by the design of the device, and thus, is highly reproducible. While it is well accepted that leukocyte migratory behaviour may be dependent on the context of the local microvascular and tissue environment [30] , [39] , this important pathophysiological issue is not acknowledged in data obtained from traditional assays such as Dunn and Zigmond chambers [11] , [12] , micropipette techniques [13] as well as the majority of microfluidic cell migration platforms [17] , [19] where cells migrate on flat surfaces. In our device, leukocytes migrate in conditions of mechanical confinement inside narrow side microchannels. Narrow channels recapitulate environmental cues that neutrophils and lymphocytes encounter in vivo within the extracellular matrix, where leukocytes move between cells within tissues [29] , [40] , [41] , [42] , [43] , [44] , [45] . Confining the cells to microchannels has the added advantage of allowing for more precise measurements of migratory speed and DP [14] , [22] , [23] , [24] . The patterns of cell migration through these microchannels are distinct from the more ‘noisy’ patterns of cells on two-dimensional flat surfaces encountered in traditional cell migration assays [11] , [12] , [13] . Microfabricated channels are also more precise and better suited for precise measurements of cell migration than 3D gels, which have heterogeneous pore size, tortuous neutrophils paths, and low orientation bias [46] . Furthermore, advantages of confining cells in microchannels are demonstrated by the results of our experiments using channels of different sizes. We found that cells within 6 × 6 μm channels display faster migratory speed and higher DP than 50 × 6 μm channels, and that cells are able to reverse their direction inside the smaller channels in the case of low-persistence migration patterns. The higher DP and speed through narrower channels is likely a result of the mechanical confinement. Similar differences in speed and persistence have been reported for epithelial cells in channels of various sizes [47] . Differences in the chemokine gradients in channels of different sizes are unlikely to contribute to the observed disparity since we found cell migration characteristics through narrow channels to be similar to wider channels in the presence of various chemokine concentrations and various gradients corresponding to these. A key finding enabled by our devices is that C5a and IL-8, two well-established chemoattractants [25] , [31] , [32] , [48] , [49] , [50] , elicit simultaneous neutrophil migration both towards and away from the chemokine gradient. This finding challenges the current views of neutrophil attraction by C5a [26] and provides a more nuanced view for the responses of neutrophils during inflammation. It suggests that complement activation and production of C5a not only serve as chemoattractants, but also activate and disperse neutrophils at the site of inflammation. While C5a is also capable of activating neutrophils to release enzymes and oxidants [51] , the bi-directional migration patterns induced by localized release of C5a could explain the more extensive tissue damage in rapidly evolving disease states [32] . In addition, while the chemoattractive and chemorepulsive actions of IL-8 have been previously reported [8] , they appear to be specific for conditions of high gradient steepness and high average chemokine concentrations. What we find is that bi-directional migration patterns are preserved even when IL-8 concentrations change. The differences between our findings and previously reported studies may be due to differences in the cell microenvironment corresponding to differences in experimental settings, such as mechanical confinement versus flat surfaces, no-flow versus shear stress, and so on. This possibility is supported by the dissimilarities in the neutrophil migration speed, 2–7 μm min −1 on flat surfaces versus 18.6–21.5 μm min −1 in channels [8] , and other differences in responses in the two experimental systems. Another possibility for the bi-directional migratory responses to C5a and IL-8 is that cells respond to chemokine stimulation in a more stochastic manner than previously appreciated. This possibility is supported by the finding that sorted populations of IL-8R hi and IL-8R lo populations show equivalent bi-directional migratory responses to IL-8. We suggest that homogenous levels of individual chemokine receptor in neutrophil subpopulations [52] , [53] do not necessarily result in a homogenous migratory response. Furthermore, our results using sorted CD177 hi and CD177 lo subpopulations showed bi-directional migratory patterns in response to gradients of either C5a or IL-8. The bi-directional effect is not specific to cell confinement, since neutrophils migrate in equal proportions towards and away from gradients in channels wider than the cells, when cells get less physical guidance. Collectively, these results indicate that bi-directional response(s) are more common than previously reported and warrant further investigation. We also suggest that bi-directional migratory behaviour may be relevant to the different strategies that neutrophils employ in the course of encountering pathogens in vivo. For example, chemoattractants, such as fMLP or LTB4, may guide neutrophils over large distances towards sites of inflammation (for example, neutrophil swarming enhancement by LTB4 (ref. 33 )), whereas C5a and IL-8 activate neutrophils in a manner that serves to enhance motility and thus allow for dispersal of subsets of cells at the site of inflammation. Future studies to better understand this bi-directional migration paradigm could include technologies that transfer individual cells from the microfluidic devices to surface cytometry systems after the migration patterns have been measured. Unfortunately, this approach requires significant technological advances that are not available today. Similarly, we found that high concentrations of SDF-1 also elicit simultaneous CD3+ and CD4+ T lymphocyte migration both towards and away from the chemokine. Again, previous reports recognized the ability of SDF-1 to repel lymphocytes [9] , [43] , [54] , but our new device reveals that this occurs simultaneously with a notable chemoattractant effect. Furthermore, we show that CD4+ T lymphocytes have a migratory signature that is similar to pooled populations of CD3+ T cells, suggesting that the attracted and repulsed cells are not different subpopulations. One interesting finding is that few lymphocytes migrate persistently towards or away from SDF-1, while the majority of the cells switch directions rather frequently. It is thus important to take into account that when measuring leukocyte migration, there is sufficient time and space for the cells to reverse their direction. This pattern of bi-directional migration would be difficult to capture in a Boyden chamber or in a transwell assay, where cells initially migrating through the membrane are not able to reverse direction. In this manner, experimental data could be interpreted as persistent attraction of the cells due to the rectifying effect of the membrane and only corrected in checkerboard assays. Overall, according to the results of our study, the patterns of migration induced by SDF-1, as well as C5a and IL-8, may be best classified as ‘dispersive’ and appropriate for ‘patrolling’ a tissue; they do not function as molecules that simply direct chemical migration towards a precise target. Our observation that Slit2 inhibits the migration of human neutrophils and HL-60 cells is consistent with previous reports [38] , [55] , [56] . In addition, measurements using our platform suggest that Slit2 reduces the fraction of cells responding to the chemoattractant, without altering migratory speed or migratory persistence and without delaying the migratory response. This signature effect of Slit2, modulating the numbers of responsive cells but not their migration phenotype, may have important anti-inflammatory implications. In summary, our characterization of leukocyte migration in microfluidic devices reveals signatures that are complex and specific to each leukocyte–chemokine combination. These signatures are not fully appreciated using traditional leukocyte chemotaxis tools and assays, which focus mostly on the analysis of chemoattraction. Other patterns of migration that coexist with chemoattraction are usually ignored but may hold valuable clues for the activity of the chemokines in health and disease. We suggest that the analysis of migration signatures based on the direction, speed, persistence and percentage of moving cells, could have broad implications for advancing our understanding of inflammatory responses, and could accelerate the screening for new therapeutics to modulate acute and chronic inflammation. Microfluidic devices The microfluidic devices were manufactured using standard microfabrication techniques. Briefly, three layers of negative photoresist (SU8, Microchem, Newton, MA), the first 3 μm thin, the second 6 μm thick and the third 50 μm thick were patterned on a silicon wafer by sequentially employing three photolithography masks and processing cycles according to the instructions from the manufacturer. The wafer with patterned photoresist was used as a mould to produce PDMS (Polydimethylsiloxane, Fisher Scientific, Fair Lawn, NJ) parts, which were then bonded irreversibly to standard glass slides (75 × 25 mm, Fisher Scientific). Neutrophil and T lymphocyte isolation For neutrophil isolation, human peripheral blood samples from healthy volunteers, aged 18 years and older, were purchased from Research Blood Components, LLC. Peripheral blood was drawn in 10-ml tubes containing a final concentration of 5 mM EDTA (Vacutainer; Becton Dickinson). Nucleated cells were isolated using a HetaSep gradient, followed by the EasySep Human Neutrophil Enrichment Kit (STEMCELL Technologies, Vancouver, Canada) according to the manufacturer’s protocol. T lymphocytes were isolated from human blood samples also obtained from healthy volunteers consented in accordance with IRB approval by Children’s Hospital Boston. PBMC were collected from peripheral blood by gradient centrifugation (2,200 r.p.m. for 30 min) using Ficoll (GE Healthcare, Waukesha, WI). CD3+ T cells were positively isolated from PBMC using magnetic beads (Dynabeads FlowComp Human CD3 isolation kit, Invitrogen, Carlsbad, CA) according to the manufacturer’s protocol, yielding bead-free cells. The purity of isolated CD3+ cells was determined using flow cytometry and found to be better than 98%. CD4+ T cells were isolated by negative selection from PBMC using magnetic beads (RosetteSep Human CD4+ T-Cell Enrichment Cocktail, STEMCELL Technologies, Vancouver, Canada) according to the manufacturer’s protocol. Cell culture and migration buffers HL-60 cells (CCL-240, ATCC, Manassas, VA) were cultured at 37 °C in 5% CO 2 in Iscove’s Modified Dulbecco’s Medium (IMDM, ATCC, Manassas, VA) containing 20% FBS (Sigma-Aldrich, St Louis, MO) and differentiated to neutrophil-like cells by DMSO-induced differentiation for a period of 5 days. Cells were sub-cultured every third day to a density of 1 × 10 6 cells ml −1 . During migration assays, neutrophils were suspended in a buffer of 0.2% human serum albumin (Sigma-Aldrich) in Hanks Buffered Salt Solution (ATCC, Manassas, VA). T lymphocytes were suspended in RPMI 1640 media (Cambrex, Charles City, IA) containing 10% fetal bovine serum, 2 mM L -glutamine, 100 U ml −1 penicillin/streptomycin (Gibco-Invitrogen), 1% sodium bicarbonate and 1% sodium pyruvate (Cambrex). Chemotaxis measurements The microfluidic device was primed 15 min before cell loading with chemokines: fMLP (Sigma-Aldrich, St Louis, MO), leukotriene B4 (LTB4, Cayman Chemicals, Ann Arbor, MI), IL-8, C5a (R&D Systems, Minneapolis, MN), or SDF-1 (Peprotech Inc, Rocky Hill, NY) were diluted in complete media. Slit2 (Abcam, Cambridge, MA) was employed alone or in combination with other chemokines. A blunt needle connected to the inlet of the device served as a loading reservoir. 20 μl of the solution of desired chemokines mixed with 100 nM human fibronectin (0.1%, Sigma-Aldrich) was added to the needle reservoir. A 1 ml syringe (Hamilton Syringes, Reno, NV) was then connected to the needle. By applying pressure through the syringe, the solution was instilled into the device. Time was allowed for the air initially trapped in dead-end chambers to diffuse out through the PDMS, under the pressure from the syringe while the outlet port was blocked. After 15 min, another 1 ml syringe filled with 100 μl cell media solution was applied to a new needle connected to the inlet, and used to wash the chemokine solution from the cell-loading chamber and migration channels. After careful washing, 10 μl of cell solution containing 2 × 10 5 cells was added to the needle reservoir and then gently delivered into the cell-loading chamber. The dead-end reservoirs were primed at the beginning of each experiment and served as the source of chemoattractant. The reservoirs are connected to the main channel through channels that have a much higher resistance than the rest of the device, such that immediately after the washing step, a chemokine free environment is created in the main channel and the buffer channel. The passive diffusion of chemoattractant from the reservoirs into the main channel creates a gradient where the highest concentration is in the reservoir and the lowest concentration is in the main channel as reported [14] . A second gradient forms between the main channel and the buffer channel by diffusion, with the higher concentration in the main channel. Cell migration was recorded using time-lapse imaging on a fully automated Nikon TiE microscope ( × 10 magnification) with a biochamber heated to 37 °C with 5% carbon dioxide gas, for 3 (HL-60 and neutrophils) or 8 h (T lymphocytes). Cell displacement was tracked manually using ImageJ (NIH). We tracked and defined a cell as a migrating cell when it entered a migration channel by at least one cell length. For neutrophils entering the narrow channels, this is ~20 μm, for lymphocytes, this length is ~10 μm. Separate experiments to characterize the formation of gradients inside the device were performed in the absence of cells, by replacing the chemoattractant with fluorescein–dextran solution (Sigma) of comparable molecular weight, and by subsequently analysing the distribution and changes in fluorescence intensity from time-lapse imaging. The migratory response of human neutrophils was studied in narrow 6 μm and wide 50 μm channels. HL-60 cells were studied in narrow 6 μm channels and T lymphocytes were studied in 10 μm channels. All channels were 6 μm in height. Wider channels optimize T lymphocytes migration, because T cells have a round and less deformable nucleus compared to neutrophils, which have a polymorph nucleus that is highly deformable, enabling them to migrate through pores of smaller sizes [29] . For these reasons, 10 μm and 6 μm wide channels were used for lymphocyte and neutrophil migration assays respectively. Analysis of cell migration Cell migration was characterized along four parameters: (1) percentage of cells migrating, (2) direction of migration, (3) speed of migration and (4) DP. The percentage of cells migrating is calculated from the number of cells migrating in each direction divided by the total amount of cells loaded in the cell-loading reservoir. The direction of migration can be either towards or away from the chemokine. Speed and DP are determined by analysing the trajectories of leukocytes moving along the channels for the following quantitative metrics: (1) relative displacement (the difference between the initial and the final cell position within the migration channel) and (2) the total distance travelled (the sum of the distances travelled in successive images) and (3) the duration of migration. Speed is determined by total distance travelled divided by the duration of migration. DP measures the persistence of migration of individual cells relative to the direction of the chemokine gradient and is calculated as relative displacement divided by total travelled distance. For cells migrating through the side channels in the direction of the chemokine reservoir DP falls between 0 and +1; in contrast, for cells migrating away from the chemokine reservoirs DP falls between 0 and −1. DP is equal to ‘1’ for cells migrating persistently toward the chemokine reservoir without changing direction and was equal to ‘−1’ for cells migrating persistently away from the chemokine reservoir, without any change in direction. DP changes for cells that make U-turns and change direction, and is equal to ‘0’ for cells that migrate back and forth through the channels and ultimately return to their initial starting position by the end of the experiment. The higher the DP, the more persistently the cells migrate in one direction. We divided individual cells into three groups (1) high persistence (DP (0.66–1) ), (2) medium persistence (DP (0.33–0.66)), and (3) low persistence (DP (0–0.33)). The BD index is the population based average migratory pattern that combines the DP and the direction of all cells. It is calculated as the sum of DP of all cells towards the chemokine plus the sum of DP of all cells migrating away from the chemokine, divided by the number of migrating cells. The measures of DP, BD index, migration speed and percentage of migrating cells were used to describe cell migratory behaviours. Cell sorting Human neutrophils were stained with FITC conjugated anti-CD177, anti-IL-8R (CD181, CXCR1, Biolegend, San Diego, CA), and either IgG1 or IgG2b (BD Pharmingen, San Jose, CA) as a control for 30 min at 4 °C and sorted on a FACSAria (BD Biosciences). Data were analysed using FlowJo Software (TreeStar, Ashland, OR). Statistical analysis For most comparisons of two experimental conditions, statistical significance was determined using the student t- test for normally distributed data and the Mann–Whitney test for data that did not have normal distribution. To compare multiple populations, we employed one-way analysis of variance with Tukey’s post hoc test. Differences were considered statistically significant when P values were less than 0.05. How to cite this article : Boneschansker, L. et al. Microfluidic platform for the quantitative analysis of leukocyte migration signatures. Nat. Commun. 5:4787 doi: 10.1038/ncomms5787 (2014).